Polytype control of spin qubits in silicon carbide Crystal defects can confine isolated electronic spins and are promising candidates for solid-state quantum information. Alongside research focusing on nitrogen-vacancy centres in diamond, an alternative strategy seeks to identify new spin systems with an expanded set of technological capabilities, a materials-driven approach that could ultimately lead to ‘designer’ spins with tailored properties. Here we show that the 4H, 6H and 3C polytypes of SiC all host coherent and optically addressable defect spin states, including states in all three with room-temperature quantum coherence. The prevalence of this spin coherence shows that crystal polymorphism can be a degree of freedom for engineering spin qubits. Long spin coherence times allow us to use double electron–electron resonance to measure magnetic dipole interactions between spin ensembles in inequivalent lattice sites of the same crystal. Together with the distinct optical and spin transition energies of such inequivalent states, these interactions provide a route to dipole-coupled networks of separately addressable spins. The search for coherently addressable spin states [1] in technologically important materials is a promising direction for solid-state quantum information science. Silicon carbide, a particularly suitable target [2] , [3] , [4] , is not a single material but a collection of about 250 known polytypes. Each polytype is a binary tetrahedral crystal built from the same two-dimensional layers of silicon and carbon atoms, but different stacking sequences give each its own crystal structure, set of physical properties and array of applications. 4H- and 6H-SiC, the most common hexagonal polytypes, are used for power and opto-electronics, and as growth substrates for graphene [5] and gallium nitride [6] . The cubic 3C-SiC can be grown epitaxially on silicon [7] and is often used in micromechanics [8] . Driven by computational [2] , [9] , [10] , [11] , electron paramagnetic resonance [9] , [10] , [12] , [13] , [14] , [15] , [16] , [17] and optical studies [3] , [12] , [13] , [18] , [19] , [20] , [21] , [22] , research into defect-based spins in SiC has also led to their increasing appreciation as candidate systems for quantum control. Our results demonstrate that despite their varying optical, electronic and structural properties, the three most common SiC polytypes all exhibit optically addressable spin states with long coherence times. These spins are localized electronic states bound to neutral divacancies [9] and related defects. Increasingly complex polytypes of SiC can host an increasing number of inequivalent defect sites–for instance, there are n inequivalent divacancy sites in n H-SiC. We measure magnetic dipole–dipole interactions between ensembles of inequivalent spins and use these interactions to infer an estimate for the degree of optical spin polarization, 35–60%, depending on the defect species. These high polarization values are an important parameter for optically addressed spin control. Moreover, as these inequivalent defect sites are separately addressable through distinct optical and spin transition energies, extending our results to the single-spin limit could lead to quantum networks of dipole-coupled spins. Optically detected spin states in SiC To generate defect ensembles in SiC, we began with semi-insulating (SI), n-type and undoped SiC substrates. In substrates with a low intrinsic defect concentration, we then used carbon ion implantation followed by an annealing process [12] designed to join vacancies into complexes (see Methods and Supplementary Note 1 ). The 3C-SiC samples consist of single and polycrystalline epitaxial films grown on silicon substrates, while the 4H- and 6H-SiC substrates are bulk single crystals. Our optically detected magnetic resonance (ODMR) measurements show that all three measured polytypes host a number of optically addressable defect spins. These ODMR measurements rely on spin-dependent optical cycles both to polarize spins with laser illumination and to measure those spin states through changes in the photoluminescence (PL) intensity. We focus on defect optical transitions with zero-phonon lines in the 1.08–1.2 eV range [12] , [23] . These can be observed as peaks in the PL spectrum when the samples are illuminated with higher energy laser excitation ( Fig. 1a ). In addition to these sharp peaks, much of the PL from these defects is emitted in broad phonon sidebands at lower energies, which we also collect. 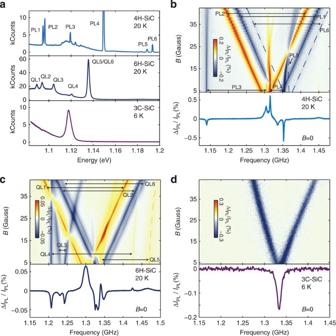Figure 1: Optical and spin transition spectra in the three most common SiC polytypes. (a) Optical spectrum of as-grown SI 4H-SiC,12C-implanted SI 6H-SiC and12C-implanted n-type 3C-SiC. (b) ODMR spectrum of SI 4H-SiC as a function ofBparallel to thecaxis (upper) and atB=0 (lower), showing six pairs of spin resonance lines. PL5 and PL6 appear faintly and are highlighted with dashed lines. (c) ODMR spectrum of SI 6H-SiC as a function ofcaxisB(upper) and atB=0 (lower), with a dashed lined highlighting the higher frequency QL5 resonance. (d) ODMR spectrum of 3C-SiC as a function of [100]-orientedB(upper) and atB=0 (lower). The 3C-SiC spins and thec-axis-oriented defects in the hexagonal polytypes (PL1, PL2, PL6, QL1, QL2 and QL6) have C3νsymmetry. The others (PL3, PL4, PL5, QL3, QL4 and QL5) are oriented along basal planes, resulting in the lower C1hsymmetry and non-degenerate spin transitions atB=0. Figure 1: Optical and spin transition spectra in the three most common SiC polytypes. ( a ) Optical spectrum of as-grown SI 4H-SiC, 12 C-implanted SI 6H-SiC and 12 C-implanted n-type 3C-SiC. ( b ) ODMR spectrum of SI 4H-SiC as a function of B parallel to the c axis (upper) and at B =0 (lower), showing six pairs of spin resonance lines. PL5 and PL6 appear faintly and are highlighted with dashed lines. ( c ) ODMR spectrum of SI 6H-SiC as a function of c axis B (upper) and at B= 0 (lower), with a dashed lined highlighting the higher frequency QL5 resonance. ( d ) ODMR spectrum of 3C-SiC as a function of [100]-oriented B (upper) and at B =0 (lower). The 3C-SiC spins and the c -axis-oriented defects in the hexagonal polytypes (PL1, PL2, PL6, QL1, QL2 and QL6) have C 3 ν symmetry. The others (PL3, PL4, PL5, QL3, QL4 and QL5) are oriented along basal planes, resulting in the lower C 1 h symmetry and non-degenerate spin transitions at B= 0. Full size image The ODMR spectra ( Fig. 1b–d ) are obtained by measuring the fractional change in PL intensity (Δ I PL / I PL ) under continuous wave laser illumination as a function of both an applied out-of-plane DC magnetic field ( B ) and the frequency ( f ) of an applied radiofrequency (RF) magnetic field. Spin flips produce a Δ I PL / I PL signature and occur when f is resonant with one of the defect’s spin transitions, which can all be tuned by varying B . The large number of observed ODMR lines demonstrates the versatility of SiC as a host for optically addressable spin states. In each polytype, wavelength-resolved ODMR measurements associate the various ODMR features with specific PL lines (see Koehl et al. [3] and Carlos et al. [13] for 4H-SiC and Supplementary Fig. S1 for 6H- and 3C-SiC). Some of the defects in 4H-SiC (PL1-PL4) have been identified as spin-1 neutral divacancies [9] . The defects responsible for the other spin transitions observed (compiled in Supplementary Table S1 ) have similar spin and optical properties to the neutral divacancies but have not been conclusively identified. Spin coherence at cryogenic and room temperatures Long-lived spin coherence, an important prerequisite for quantum information and sensing technologies, is a general feature of spins in all three polytypes. Our coherence measurements are based on standard pulsed magnetic resonance techniques including Rabi, Ramsey, Hahn echo, Carl-Purcell-Meiboom-Gill ( Fig. 2 ) and spin relaxation ( Supplementary Fig. S2 ) sequences. At 20 K, the spin relaxation times range from 8 to 24 ms. The Hahn-echo coherence times ( T 2 ) range from 10 μs to 360 μs at 20 K, depending on the substrate, with significant dependence on implantation dose and substrate doping type. The longest T 2 times we measured were in native neutral divacancies in 4H-SiC that were generated during crystal growth. 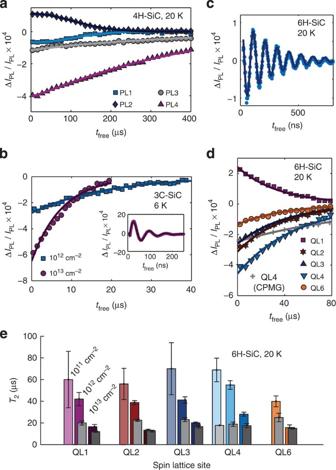Figure 2: Ensemble spin coherence at cryogenic temperatures. (a) Hahn-echo measurement of spin coherence of the neutral divacancies in as-grown SI 4H-SiC at 20 K, showingT2times of 140±5 μs (PL1), 144±3 μs (PL2), 360±20 μs (PL3) and 340±5 μs (PL4). Long Rabi pulses (150 kHz) were used to minimize decoherence from instantaneous diffusion. (b) Hahn-echo measurement of the 3C-SiC spins at 6 K, implanted with12C at doses of 1012cm−2and 1013cm−2, with respective decoherence times ofT2=24±4 μs andT2=12±1 μs. Inset: Ramsey measurement of 3C-SiC spin dephasing, showingT2*=52±3 ns. (c) Ramsey measurement at 20 K of QL4 in SI 6H-SiC implanted with12C at a dose of 1012cm−2. RF pulses were detuned from resonance by 10 MHz. The fit is to an exponentially decaying sinusoid withT2*=250 ns. (d) Hahn-echo measurement for QL1–QL6 in 1012cm−2-implanted SI 6H-SiC at 20 K, except for QL5, whose overlap with other ODMR lines atB=0 inhibited zero-field measurements. Carl–Purcell–Meiboom–Gill (CPMG) dynamical decoupling for QL4 is also shown, withTCPMG=106±2 μs. The Rabi frequencies used (2.5 MHz) are less than the inhomogeneous linewidth, resulting in roughly half of the spins being driven. (e) Comparison of 20 K Hahn-echo coherence times in n-type 6H-SiC (grey) and SI 6H-SiC (coloured) for three different12C implantation doses and spin densities. The error bars are 95% confidence intervals from exponential fits to the Hahn-echo data.B=0 for all the data in this figure. Figure 2: Ensemble spin coherence at cryogenic temperatures. ( a ) Hahn-echo measurement of spin coherence of the neutral divacancies in as-grown SI 4H-SiC at 20 K, showing T 2 times of 140±5 μs (PL1), 144±3 μs (PL2), 360±20 μs (PL3) and 340±5 μs (PL4). Long Rabi pulses (150 kHz) were used to minimize decoherence from instantaneous diffusion. ( b ) Hahn-echo measurement of the 3C-SiC spins at 6 K, implanted with 12 C at doses of 10 12 cm −2 and 10 13 cm −2 , with respective decoherence times of T 2 =24±4 μs and T 2 =12±1 μs. Inset: Ramsey measurement of 3C-SiC spin dephasing, showing T 2 *=52±3 ns. ( c ) Ramsey measurement at 20 K of QL4 in SI 6H-SiC implanted with 12 C at a dose of 10 12 cm −2 . RF pulses were detuned from resonance by 10 MHz. The fit is to an exponentially decaying sinusoid with T 2 *=250 ns. ( d ) Hahn-echo measurement for QL1–QL6 in 10 12 cm −2 -implanted SI 6H-SiC at 20 K, except for QL5, whose overlap with other ODMR lines at B =0 inhibited zero-field measurements. Carl–Purcell–Meiboom–Gill (CPMG) dynamical decoupling for QL4 is also shown, with T CPMG =106±2 μs. The Rabi frequencies used (2.5 MHz) are less than the inhomogeneous linewidth, resulting in roughly half of the spins being driven. ( e ) Comparison of 20 K Hahn-echo coherence times in n-type 6H-SiC (grey) and SI 6H-SiC (coloured) for three different 12 C implantation doses and spin densities. The error bars are 95% confidence intervals from exponential fits to the Hahn-echo data. B =0 for all the data in this figure. Full size image All three polytypes exhibit defects whose spin coherence persists up to room temperature ( Fig. 3 and Supplementary Figs S3–S5 ). In as-grown 4H-SiC, one neutral divacancy line (PL3) persists up to room temperature as well as three other ODMR lines (PL5–PL7) of unknown origin, all with T 2 =50±10 μs. Polycrystalline 3C-SiC also exhibits a state with room-temperature spin coherence, although similar states with the same zero-phonon line and ODMR transition in certain other 3C-SiC substrates that we measured did not. In 6H-SiC, the SI and n-type substrates have the same ODMR lines at 20 K, but their room-temperature ODMR signatures are substantially different from each other ( Fig. 3b ), with several additional ODMR lines in the n-type substrate that do not appear at 20 K or in the SI substrate. The presence of these coherent spin states at room temperature is a particularly promising result for spin-based sensing [24] with SiC. 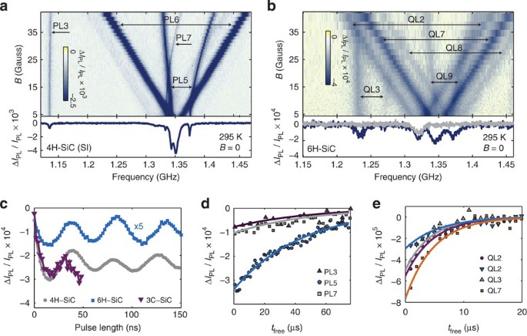Figure 3: Ensemble spin coherence at room temperature. (a) ODMR in as-grown SI 4H-SiC as a function ofB(upper) and atB=0 (lower). (b) ODMR as a function ofBin n-type 6H-SiC (upper) and atB=0 (lower) for n-type (dark blue) and SI (grey) 6H-SiC, implanted at 1013cm−2dose of12C. QL7–QL9 have reduced ΔIPLcontrast as the temperature is lowered, disappearing by 200 K. (c) Rabi driving at room temperature: PL5 in SI 4H-SiC, QL2 in SI 6H-SiC (multiplied by a factor of × 5), and the 3C-SiC spin species. (d) Hahn-echo measurements of room-temperature coherence for spin states in as-grown SI 4H-SiC. The fittedT2times are 50±30 μs (PL3), 44±2 (PL5) and 50±15 μs (PL7). (e) Hahn-echo measurement of room-temperature coherence in n-type and SI 6H-SiC, implanted at the 1013cm−2dose. The fittedT2times are 4.7±0.6 μs (purple, QL2, n-type), 5.6±1.8 μs (turquoise, QL2, SI), 4.4±1.5 μs (gray, QL3, n-type) and 4.9±0.9 μs (orange, QL7, n-type). The uncertainties are 95% confidence intervals from exponential fits to the Hahn-echo data. Figure 3: Ensemble spin coherence at room temperature. ( a ) ODMR in as-grown SI 4H-SiC as a function of B (upper) and at B =0 (lower). ( b ) ODMR as a function of B in n-type 6H-SiC (upper) and at B =0 (lower) for n-type (dark blue) and SI (grey) 6H-SiC, implanted at 10 13 cm −2 dose of 12 C. QL7–QL9 have reduced Δ I PL contrast as the temperature is lowered, disappearing by 200 K. ( c ) Rabi driving at room temperature: PL5 in SI 4H-SiC, QL2 in SI 6H-SiC (multiplied by a factor of × 5), and the 3C-SiC spin species. ( d ) Hahn-echo measurements of room-temperature coherence for spin states in as-grown SI 4H-SiC. The fitted T 2 times are 50±30 μs (PL3), 44±2 (PL5) and 50±15 μs (PL7). ( e ) Hahn-echo measurement of room-temperature coherence in n-type and SI 6H-SiC, implanted at the 10 13 cm −2 dose. The fitted T 2 times are 4.7±0.6 μs (purple, QL2, n-type), 5.6±1.8 μs (turquoise, QL2, SI), 4.4±1.5 μs (gray, QL3, n-type) and 4.9±0.9 μs (orange, QL7, n-type). The uncertainties are 95% confidence intervals from exponential fits to the Hahn-echo data. Full size image Coherent spin interactions Ultimately, many spin-based quantum technologies will require not only separately addressable spins with long coherence times but also a means of coupling these spins together. Patterned ion implantation has generated individual and strongly coupled nitrogen-vacancy (NV) centres in diamond [25] . We have also patterned spin ensembles in SiC, using ion implantation through poly-(methyl-methacrylate) (PMMA) apertures ( Fig. 4a ; Supplementary Fig. S6 ). Though these are not individual spins, this patterning demonstration shows promise for spatially engineering SiC defects. As optical wavelengths significantly exceed the length scale required for strong magnetic coupling between single dipoles (<30 nm for diamond NV centres [25] ), scaling up a dipole-coupled spin network is a significant challenge. Silicon carbide defects in inequivalent lattice sites have distinct RF and optical transition energies, giving complex polytypes of SiC with many inequivalent defect species the possibility of hosting many separately addressable spins in a single confocal volume ( Fig. 4b ). 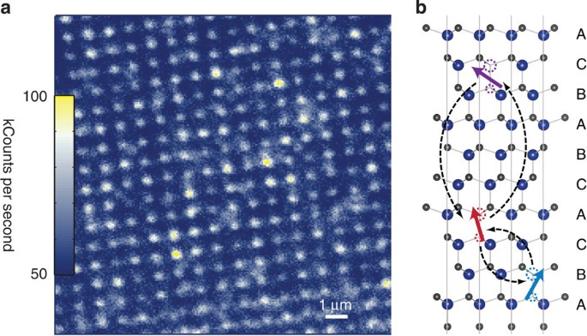Figure 4: Patterned SiC spins and illustration of dipole-coupled spins. (a) Implanted spin ensembles in n-type 4H-SiC through a PMMA mask with 50 nm holes, using 10 keV energy12C ions at a 1013cm−2dose. Additional characteristics of these implanted spins are given inSupplementary Fig. S6. (b) Illustration of dipole-coupled spin network in 6H-SiC in which each spin has a unique orientation and optical/ODMR signature. The three spins shown here are the (hh) divacancy (turquoise), (k1k1) divacancy (purple) and (k2k2) divacancy (red). Figure 4: Patterned SiC spins and illustration of dipole-coupled spins. ( a ) Implanted spin ensembles in n-type 4H-SiC through a PMMA mask with 50 nm holes, using 10 keV energy 12 C ions at a 10 13 cm −2 dose. Additional characteristics of these implanted spins are given in Supplementary Fig. S6 . ( b ) Illustration of dipole-coupled spin network in 6H-SiC in which each spin has a unique orientation and optical/ODMR signature. The three spins shown here are the (hh) divacancy (turquoise), (k 1 k 1 ) divacancy (purple) and (k 2 k 2 ) divacancy (red). Full size image As a step towards independently addressable dipole-coupled spins, we measure dipole–dipole spin interactions between inequivalent defect ensembles. The study of these interactions also provides valuable information about the spin density and optical polarization in these defect states. Our measurements use double electron–electron resonance [26] (DEER) to flip the spin of one spin ensemble (the ‘drive’ species), while the resulting change in the Larmor precession rate of another ensemble (the ‘sense’ species) is measured. We focused on 6H-SiC for these measurements, which when implanted, had higher spin densities than in our 4H-SiC substrates, and higher DEER-coupling strengths. The change in precession rate (Δ f ), a measure of the average dipole-coupling strength, is experimentally observed as an additional phase (Δ θ free ) acquired by the sense species over the free precession segment of a Hahn-echo measurement ( Fig. 5a ). These parameters are related by , where t pulse is the delay of the drive pulses relative to the center of the Hahn-echo sequence. This pulse sequence is designed to refocus the sense spins due to all magnetic fields except those due to drive species spin flips. When we drive Rabi oscillations on the drive species, we simultaneously observe DEER oscillations in Δ θ free of the sense spins ( Fig. 5b ). 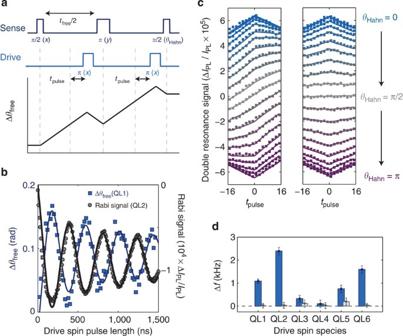Figure 5: Magnetic dipole-coupled spin ensembles in 6H-SiC. (a) Pulse scheme for DEER measurements. Asπpulses flip the orientation of the drive species spins, the sense species accumulates an extra phase (Δθfree) over a Hahn-echo sequence. (b) Varying the pulse duration of the drive spins (QL2) generates Rabi oscillations (right axis) and an oscillation in the DEER signal (left axis) corresponding to the sense spin species (QL1) acquiring Δθfree. The Rabi data are fitted according to an erfc-decaying sinusoid30and Δθfreeis fitted to a multiple of this function. (c) DEER signal, applying twoπpulses to the drive species and varyingθHahnandtpulse. The left data set is when the drive spins are polarized, and the right data set is for unpolarized spins, for which Δfvanishes. The data at differentθHahnare not artificially offset. The solid lines are global fits to Equation 1. (d). Fitted Δffor the six spin orientations, when the drive-spin species is polarized (blue) and unpolarized (grey). The sense species is QL1 for all these data, except when QL1 is driven, in which case it is QL2.B=64 G andtfree=32 μs andT=20 K for all the data inFig. 5. Figure 5: Magnetic dipole-coupled spin ensembles in 6H-SiC. ( a ) Pulse scheme for DEER measurements. As π pulses flip the orientation of the drive species spins, the sense species accumulates an extra phase (Δ θ free ) over a Hahn-echo sequence. ( b ) Varying the pulse duration of the drive spins (QL2) generates Rabi oscillations (right axis) and an oscillation in the DEER signal (left axis) corresponding to the sense spin species (QL1) acquiring Δ θ free . The Rabi data are fitted according to an erfc-decaying sinusoid [30] and Δ θ free is fitted to a multiple of this function. ( c ) DEER signal, applying two π pulses to the drive species and varying θ Hahn and t pulse . The left data set is when the drive spins are polarized, and the right data set is for unpolarized spins, for which Δ f vanishes. The data at different θ Hahn are not artificially offset. The solid lines are global fits to Equation 1. ( d ). Fitted Δ f for the six spin orientations, when the drive-spin species is polarized (blue) and unpolarized (grey). The sense species is QL1 for all these data, except when QL1 is driven, in which case it is QL2. B =64 G and t free =32 μs and T =20 K for all the data in Fig. 5 . Full size image To measure both Δ f and the decoherence rate of the sense spins due to drive-spin flips ( τ ), we vary both t pulse and the phase of the final π /2 pulse in the sense spin Hahn-echo sequence ( θ Hahn ). The resulting data ( Fig. 5c , left) are well fit by: For the data at θ Hahn = π /2, the coherent coupling term becomes in equation (1), providing a sensitive measure of Δ f, while the data at θ Hahn =0 and θ Hahn = π are dominated by the decoherence term, giving a more accurate measure of τ . The globally fitted values of Δ f for various drive-spin ensemble species ( Fig. 5d and Supplementary Fig. S7 ) show that the c -axis-oriented spins (QL1, QL2 and QL6) exhibit Δ f values in the single kHz range. The lower symmetry of the basal-oriented spins (QL3–QL5) results in eigenstates with smaller magnetic moments, reducing Δ f for these species ( Supplementary Note 2 ). We also repeated this experiment with the pulse sequence shown in Fig. 5a modified by the addition of a depolarizing π /2 pulse, which is applied to the drive spins before the sense spins’ Hahn-echo sequence. In this case, because the π pulses applied to the drive-spin population no longer cause a net change in magnetization, Δ f vanishes ( Fig. 5c , right). Additionally, when the drive spins are depolarized, τ increases slightly. When QL1 is the sense species and QL2 is the drive species, τ changes from 89±3 μs (polarized QL2) to 96±3 μs (unpolarized QL2). The decoherence characterized by τ , known as instantaneous diffusion, arises from two effects. The first (and dominant) of these is microscopically inhomogeneous dipole-coupling strengths between randomly located individual spins, resulting in a distribution of coupling strengths, whose average is Δ f . This distribution causes ensemble dephasing of the sense species when the drive species is flipped. The second effect is a macroscopically inhomogeneous magnetization field due to the spatial structure of the optically polarized volume of spins. The result of this effect is a slightly longer τ when the spin bath is depolarized, consistent with the data. The analysis of these data is complicated by the dynamics of discretely interacting spins in a polarized spin bath ( Supplementary Note 3 ). Nevertheless, the standard quasi-static statistical model relating instantaneous diffusion to spin density [26] , [27] provides a guide for analysing the DEER results. On the basis of this model, we use τ for the unpolarized spin bath to infer that the spin densities of the three c -axis spin species (QL1, QL2 and QL6) range from 7–11 × 10 15 spins cm −3 . Because Δ f is proportional to the magnetic field generated by the drive-spin ensemble, which in turn is proportional to the product of spin density and optical polarization, we can use the measured Δ f and the calculated spin density to infer the degree of optical spin polarization. For the three c -axis spins, our DEER results lead to a high average optical spin polarization that ranges from 35% to 60%, depending on the defect species. Because of the inhomogeneous spatial profile of the optical illumination and collection areas in our measurements, the full optical polarization is likely to be even higher. SiC spins are compelling analogues of diamond NV centres, with complementary properties and many unique prospects. Our demonstration that crystal polymorphism can be used to engineer new spin centres relies on SiC being a polymorphic material, a degree of freedom that is unavailable in diamond. In the future, established doping and epitaxial growth processes in SiC could lead to electronic interfaces with defect spins embedded in transistors and optoelectronic devices. Furthermore, due to its availability as a single-crystalline epitaxial film on silicon, the 3C polytype provides an excellent platform for hybrid quantum systems with photonic [28] and mechanical [29] degrees of freedom. Combining this sophisticated semiconductor technology with the versatility of coherent spin control in SiC stands to be an exciting route for solid-state quantum information. Generation of defects The 4H-SiC and 6H-SiC substrates used in this work include: a) n-type 4H-SiC, b) high-purity SI 4H-SiC, c) n-type 6H-SiC and d) SI 6H-SiC. Substrates a, b and c were purchased from Cree, Inc, while d was purchased from II-VI, Inc. The SI 4H-SiC contains a significant density of neutral divacancy spins as grown, and the data in Figs 1 , 2a and 3 used that material without modification. Defects in the other substrates were generated by an ion implantation process consisting of 190 keV 12 C ion implantations at doses of 10 11 , 10 12 and 10 13 cm −2 , with a 7-degree tilt to minimize ion channelling effects. After ion implantation, the samples were annealed at 900 °C for 30 min in Ar, a process designed to allow vacancies to diffuse and aggregate into pairs and vacancy complexes [12] . We estimate a 5% creation efficiency of fluorescent defects, defined as the number of created defects per implanted 12 C ion at 190 keV ( Supplementary Note 1 ). For the n-type substrates, ion implantation with 12 C can compensate the n-type doping. Throughout the text, our labelling of substrate doping types refers to the as-grown substrates, not to the semiconductor characteristic after implantation. The 3C-SiC substrates used in this work consisted of [100] oriented epitaxial layers grown on [100] silicon substrates. The 3C-SiC substrates measured in Figs 1 and 2 were 3.85-μm-thick films and were obtained from Novasic. The substrates measured in Fig. 3 were grown at Case Western Reserve University and consisted of 1.5–2 μm thick polycrystalline films. Neither film was intentionally doped but both showed n-type behaviour. All samples were implanted with 190 keV 12 C at doses of 10 12 or 10 13 cm −2 with a 7-degree tilt. The samples were then annealed at 750 °C for 30 min in Ar. The patterned defects in Fig. 4a were generated by ion implantation at a lower energy (10 keV 12 C ions at a dose of 10 13 cm −2 ), which makes the 170-nm-thick PMMA a more effective ion mask. The PMMA mask used for the sample in Fig. 4b consisted of 50-nm apertures patterned by electron beam lithography. Optically detected magnetic resonance For our ODMR measurements, the laser excitation was higher energy than the defects’ zero-phonon lines, within their absorption sidebands. For the 4H- and 6H- substrates in Figs 1 , 2 , 3 , 4 , the laser energy was 1.45 eV (853 nm), with 16 mW of power reaching the sample. For the 3C-SiC data in Figs 1d and 2b , the laser energy was 1.33 eV (930 nm), and the power was 23 mW at the sample. For the double resonance data in Fig. 5 , the laser energy was 1.27 eV (975 nm), with 60 mW reaching the sample. The laser excitation was gated with acousto-optical modulators and the fluorescence was collected using one of four detectors: a) a Thorlabs Femtowatt InGaAs photoreceiver (PDF10C), b) a Newport InGaAs photoreceiver (2011-FS), c) a Princeton instruments liquid-nitrogen cooled InGaAs camera attached to an Acton Spectrometer (2300i) and d) a Scontel superconducting detector (LTD 24/30-008). The samples were mounted on top of 0.5- to 2-mm RF strip lines [3] . For the 3C-SiC, ring-shaped RF waveguides fabricated on chip were also used [3] . These sample/waveguide assemblies were then mounted in optical cryostats with RF access. The RF signals were generated by two signal generators (Agilent E8257C or Rohde & Schwarz SM300 vector source) whose outputs were gated using RF switches (MiniCircuits ZASWA-2-50DR+) for pulsed experiments. These signals were then combined, amplified to peak powers as high as 25 W (Amplifier Research 25S1G4A and Mini-Circuits ZHL-30W-252-S+), and sent to wiring in the cryostat connected to the waveguides and striplines. The RF and optical pulses were gated with pulse patterns generated by either a digital delay generator (Stanford Research Systems DG645), Pulse Pattern Generator (Agilent 81110A) or arbitrary waveform generator (Tektronix AWG520). The phase of the Rohde & Schwartz signal was also controlled by the AWG520. The ODMR measurements in this paper were all taken using lock-in techniques, in which an RF pulse was alternatively gated on and off ( Figs 1 and 3a–c ) or the phase of one of the pulses was alternatively gated by 180° using IQ modulation ( Figs 2 , 3d , e and ). We used a 20-Hz software lock-in technique [3] ( Figs 1 , 2 , 3 ) and a hardware lock-in at frequencies up to 200 kHz ( Fig. 5 ) to accommodate the bandwidths of the Thorlabs and Newport photoreceivers, respectively. Because the PL spectra of the various divacancy orientations have overlapping phonon sidebands, these measurements collected I PL from all defect orientations at once. This procedure reduced the normalized Δ I PL / I PL signal but prevented defect PL from being rejected. The measured Δ I PL / I PL values are additionally reduced from their ideal values both by extra fluorescence from the SiC samples (notably Vanadium impurities in the SI 6H-SiC) and by long fluorescence collection times. To achieve high optical spin polarization, we used long optical pulses (20–100 μs) in our measurement cycles. Because the timescale of optical polarization was faster than the bandwidth of most of our detectors, we did not gate the fluorescence collection. Therefore, much of the PL collected was from defect spins already polarized earlier in the pulse. Fast and gated fluorescence detection would lead to significantly higher Δ I PL / I PL values. How to cite this article: Falk, A. L. et al. Polytype control of spin qubits in silicon carbide. Nat. Commun. 4:1819 doi: 10.1038/ncomms2854 (2013).